Metabolic modelling reveals the specialization of secondary replicons for niche adaptation inSinorhizobium meliloti The genome of about 10% of bacterial species is divided among two or more large chromosome-sized replicons. The contribution of each replicon to the microbial life cycle (for example, environmental adaptations and/or niche switching) remains unclear. Here we report a genome-scale metabolic model of the legume symbiont Sinorhizobium meliloti that is integrated with carbon utilization data for 1,500 genes with 192 carbon substrates. Growth of S. meliloti is modelled in three ecological niches (bulk soil, rhizosphere and nodule) with a focus on the role of each of its three replicons. We observe clear metabolic differences during growth in the tested ecological niches and an overall reprogramming following niche switching. In silico examination of the inferred fitness of gene deletion mutants suggests that secondary replicons evolved to fulfil a specialized function, particularly host-associated niche adaptation. Thus, genes on secondary replicons might potentially be manipulated to promote or suppress host interactions for biotechnological purposes. The last years have witnessed a growing attention towards the ecological and evolutionary implication of the multiple replicon bacterial genome [1] , [2] , [3] , [4] that is present in about 10% of sequenced bacterial genomes [1] . This genome architecture is common in the proteobacterial species that interact with a host and are of importance to the human population [1] , [2] , including crop plant symbionts (for example, Sinorhizobium and Rhizobium ), plant pathogens (for example, Agrobacterium ), and animal and human pathogens (for example, Brucella , Burkholderia and Vibrio ). As the bacterial genome is non-randomly organized [5] , it is proposed that this genome organization was shaped by selective pressures to facilitate improved host interactions and niche adaptation. Though it is well established that secondary replicons often carry genetic determinants essential to colonize a novel environment, for example, virulence or symbiotic genes, such genes often account for only a small proportion of these replicons [6] , [7] . The majority of the genes on a secondary replicon are not directly essential to colonize a specific environment, and the adaptive function of these genes and why they are localized on a secondary replicon remains unclear. Several recent studies have provided evidence consistent with the secondary replicons in a multipartite genome encoding environment-specific fitness promoting but non-essential functions [3] , [4] , [8] , [9] , [10] , [11] , [12] . However, none of these studies demonstrated that secondary replicons indeed carry environment-specific fitness determinants, thus serving as reservoirs for niche-specific functions. Sinorhizobium meliloti is a N 2 -fixing endosymbiont of legume species that has recently become a model organism for the study of bacterial multipartite genome function and evolution. All sequenced S. meliloti genomes contain at least three large replicons (the primary chromosome, the pSymB chromid and the pSymA megaplasmid), with some strains hosting additional small accessory plasmids [3] , [13] , [14] . S. meliloti experiences a complex life cycle and successfully colonizes three distinct niches. Two of these niches are bulk soil and rhizosphere soil (that is, the soil directly influenced by the plant root system), which are quite different environments, with the rhizosphere generally considered to be a nutritionally richer environment due to plant root exudates [15] . The third niche inhabited by S. meliloti is the legume root nodule. S. meliloti can induce root nodule formation in certain legumes and within nodules the bacteria differentiate into N 2 -fixing bacteroids. Manipulation and optimization of this agriculturally and ecologically important symbiosis is an ultimate goal of the rhizobial research community [16] , [17] , [18] . Effectively doing so will require a complete understanding of the evolution [18] , genetics [6] and the metabolism of the organism in both rhizosphere and nodule environments, as well as the corresponding metabolic shifts. Here we combine a genome-scale metabolic network reconstruction of the S. meliloti genome, flux balance analysis (FBA), and growth phenotype data for 11 large-scale S. meliloti deletion mutants to examine the metabolic changes accompanying the shifts between bulk soil, rhizosphere and nodule environments. We use an in silico approach to predict the phenotypes resulting from the deletion of 1,575 S. meliloti metabolic genes, estimate the fitness contribution of each replicon within each environment, and thus provide insight into the evolution of multipartite genomes. Reconstruction of a S. meliloti genome-scale metabolic model As described in the Supplementary Methods , an in silico representation of the metabolism of S. meliloti was developed, and the final model that was termed iGD1575 contained 1,575 genes, 1,825 reactions and 1,579 metabolites. 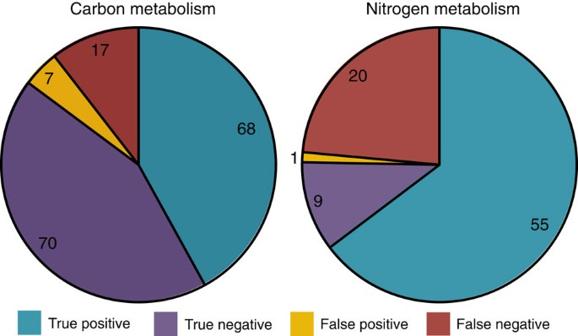Figure 1: Agreement between experimental andin silicometabolic capabilities ofS. meliloti. True positives, growth was observed experimentally andin silico. True negatives, growth was not observed experimentally orin silico. False negatives, compounds that support growth experimentally but notin silico. False positives, compounds that support growthin silicobut not experimentally. The complete set of compounds and growth predictions can be found inSupplementary Data 1. iGD1575 accounts for 25.4% of the protein-coding genes in the S. meliloti genome, and the other main features of the model are listed in Table 1 . Cluster of Orthologous Gene (COG) analyses confirmed that the gene functional biases of each replicon are accurately represented in iGD1575 ( Supplementary Fig. 1 ) [12] , [13] . The iGD1575 model encompasses 529 of the 565 genes present in iHZ565, a previously reported S. meliloti small metabolic model [19] . The remaining 31 genes were not added to iGD1575 as experimental data were inconsistent with their annotation, we felt their annotation too general to have high confidence in the enzymes’ substrates/products, or the associated reaction involved a metabolite not present in any other reaction in the model and thus the reaction would never carry flux in FBA ( Supplementary Table 1 ). Comparison of the number of genes in iGD1575 to that of other available rhizobial and non-rhizobial models [19] , [20] , [21] , [22] showed that iGD1575 is currently one of the largest metabolic reconstruction of a bacterial genome. In addition, iGD1575 is the first metabolic model capable of representing the metabolism of both a symbiotic and free-living rhizobial cell. Table 1 Summary of the main properties of iGD1575. Full size table Quantitative validation of iGD1575 Previous work [23] has shown that S. meliloti transports glucose into the cell at a rate of 2.41 mmol h −1 per g cellular dry weight. When glucose is provided to the iGD1575 model as the sole carbon source at the experimentally determined rate, a specific growth rate of 0.325 h −1 is predicted, which is consistent with our experimentally derived growth rate of 0.313 h −1 (s.d. 0.002) for S. meliloti grown with glucose. Similarly, it has been shown [24] that S. meliloti transports succinate into the cell at a rate of 6.252 mmol h −1 per g protein. Providing succinate as the sole source of carbon to iGD1575 at the experimentally determined value led to a predicted specific growth rate of 0.279 h −1 , similar to the experimentally derived growth rate of 0.254 h −1 (s.d. 0.025) for S. meliloti grown with succinate. Measuring the amount of phosphate remaining in the spent growth media following growth of S. meliloti indicated that 63.7 (s.d. 6.7) and 39.8 μM (s.d. 1.5) of phosphate was used per mM of glucose and succinate, respectively. These experimental values are relatively consistent with the phosphate usage values predicted by iGD1575 of 72.7 and 48.5 μM per mM of glucose and succinate, respectively. Little experimental flux data has been reported for S. meliloti ; however, flux measurements for 22 central carbon metabolic reactions when S. meliloti is grown with glucose as the sole source of carbon have been reported by Fuhrer et al . [23] . Not surprisingly, the experimentally determined fluxes did not match well with the iGD1575-derived values. This is because the specific growth rate of S. meliloti was only 0.17 h −1 in the study by Fuhrer et al ., indicating that S. meliloti was grown in sub-optimal conditions that presumably effected the flux distribution. Nevertheless, if the flux through these 22 central carbon metabolic reactions in iGD1575 was set to that as experimentally determined by Fuhrer et al ., the predicted specific growth rate was reduced to 0.159 h −1 , in line with the 0.17 h −1 reported by Fuhrer et al . The good relationship between flux distribution and specific growth rate, and the strong ability of iGD1575 to predict growth rate and phosphate usage when grown with glucose or succinate, suggest that the flux distributions predicted by iGD1575 should represent quantitatively accurate estimations. iGD1575 captures the metabolic capacity of S. meliloti The ability of S. meliloti to grow with various carbon and nitrogen sources has been well studied by means of the Phenotype MicroArray (Biolog) technology [4] , [25] , [26] , [27] . These previously published studies were used to guide model expansion and refinement during the curation process. 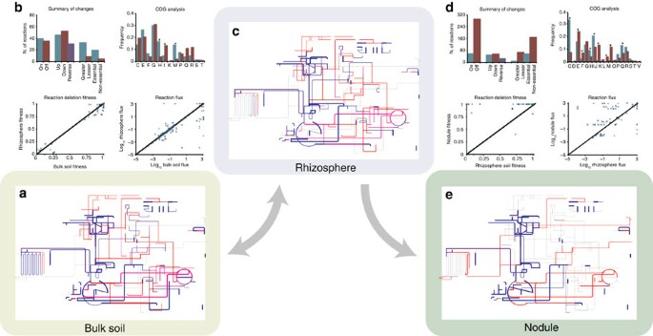Figure 2: The effect of niche conditions on the reconstructed metabolic network. Networks were visualized following optimization in (a) bulk soil, (c) rhizosphere and (e) nodule environments. Lines are colour coded based on fitness effect of deleting each reaction: blue indicates a fitness decrease <1%; dark purple indicates a fitness decrease <50%; bright purple indicates a fitness decrease >50%; and red indicates a fitness decrease >99%. Thin grey lines indicate inactive reactions. Line thickness shows the flux through each reaction on a log scale. The graphs summarize the metabolic changes detected during the (b) bulk soil to rhizosphere and (d) rhizosphere to nodule transitions. Summary of changes graphs: on and off—reactions carrying flux only in the second and first environment, respectively; up and down—reactions carrying increased flux (≥50%) in the second and first environment, respectively; reverse—reactions whose directionality is switched; greater and lesser—reactions whose removal have a greater (≥10%) fitness impact in the second and first environment, respectively; essential and non-essential—reactions essential only in the second and first environment, respectively. The nine classifications are not mutually exclusive. The reactions present in each category are described inSupplementary Data 3and4. The COG analysis graphs summarize the functional annotation of the genes associated with the reactions in the summary of changes graphs. The blue and red bars include the genes associated with the blue and red bars, respectively, in the summary of changes graphs. Asterisks indicate statistically significant changes (Pvalue <0.01) as determined by Pearson’sχ2-tests. In the reaction flux figures, each point represents the amount of flux through individual reactions in the two environments. Blue and purple symbols indicate reactions with the same or reverse directionality, respectively. The angled line indicates the position of a perfect correlation. In the reaction deletion fitness figures, each point represents the fitness of individual reaction deletion mutants in the two environments. The angled line indicates the position of a perfect correlation. Once all of the manual curation of iGD1575 was complete, FBA illustrated that the final model could accurately predict the ability of S. meliloti to produce, or not produce, biomass (as defined in Supplementary Table 2 ) on 85% (138/162) and 75% (64/85) of the tested carbon and nitrogen substrates, respectively, for which the ability of S. meliloti to utilize, or not, these compounds is known ( Fig. 1 and Supplementary Data 1 ). Most of the discrepancies between the experimental data and the iGD1575 growth prediction were false negatives (71% and 95% for growth with carbon and nitrogen substrates, respectively). These represent compounds that S. meliloti can metabolize but the model cannot use for the production of biomass, likely representing gene annotation gaps in our knowledge of S. meliloti that will serve as targets for future research. The predictive power of bacterial metabolic models reported in previous studies [28] , [29] , [30] is similar to that reported here for iGD1575. Hence, iGD1575 is at least as good as other current genome-scale metabolic reconstructions at representing the organism’s metabolic capabilities. This suggests that iGD1575 effectively captures the metabolic capacity of S. meliloti and can validly be used to model metabolism in nutritionally diverse environments. Figure 1: Agreement between experimental and in silico metabolic capabilities of S. meliloti . True positives, growth was observed experimentally and in silico . True negatives, growth was not observed experimentally or in silico . False negatives, compounds that support growth experimentally but not in silico . False positives, compounds that support growth in silico but not experimentally. The complete set of compounds and growth predictions can be found in Supplementary Data 1 . Full size image Carbon growth phenotypes of S. meliloti deletion mutants Carbon utilization phenotypes for a subset of large-scale pSymB deletion mutants [31] that cumulatively remove ∼ 1.65 Mb (98%) of pSymB ( Supplementary Fig. 2 ) were determined using PM1 and PM2A Biolog plates. This screen effectively generated a carbon utilization data set for ∼ 1,500 pSymB genes. Overall, growth was observed with 76 carbon substrates, and a total of 43 no or extremely poor growth phenotypes were observed ( Table 2 , Supplementary Figs 3 and 4 , and Supplementary Data 1 and 2 ). In the process of developing and validating iGD1575, an in silico representation of the same experiment was performed, and where possible, the model was updated to fix discrepancies between the experimental and in silico results. Following this integration of the Phenotype MicroArray data set with the metabolic reconstruction, there was very good agreement between the experimentally observed results and the in silico simulations was observed ( Table 2 and Supplementary Data 1 ). In silico simulations did not predict any ‘no growth’ phenotypes that were not experimentally observed, and 23 of the 36 (63.9%) experimentally observed phenotypes for compounds that support growth of iGD1575 were replicated in silico . Some of the discrepancies between the experimental and in silico data represent gaps in our knowledge of catabolic pathways in S. meliloti , while other phenotypes may occur for non-metabolic reasons and therefore not give a phenotype in silico . For example, the S. meliloti deletion mutant ΔB154 is more sensitive to cobalt chelation than the wild type [32] , and the lack of growth in wells with L -histidine or D -glucosamine may simply reflect cobalt chelation [33] , [34] . Table 2 Carbon utilization phenotypes observed for pSymB deletion mutants. Full size table In addition to model refinement, integrating the mutant phenotype data with iGD1575, the DuctApe software [27] , the S. meliloti genome annotation [13] and an ABC transporter induction study [35] allowed for the prediction of novel carbon catabolic loci. One example compound is the monosaccharide psicose. Our analysis suggests that psicose is transported by the SupABCD (Smb20484–Smb20487) ABC transporter, and then converted to fructose by an isomerase encoded by smb20488 . A second example is D -galactosamine, which, as elaborated on in Supplementary Note 1 , we predict is transported by the Smb21216, Smb21219–Smb21221 transporter and potentially the Smb21135–Smb21138 transporter, and then metabolized by Smb21217, Smb21218, Smb21373 and Smb21374. Rhizosphere colonization required a metabolic refinement The metabolic shifts experienced by S. meliloti during transition between bulk soil, the rhizosphere and the nodule were modelled using in silico representations of the nutritional composition of each environment. These took into account the relative ratios of each component in the different environments and the development of these environments are described in the Supplementary Methods . In the bulk soil and rhizosphere environments, the model was optimized for the production of biomass as defined in Supplementary Table 2 , whereas in the nodule environment the model was optimized for production of an effective N 2 -fixing symbiosis as defined previously [19] . The optimal flux patterns in each of the three niches were obtained using FBA and visualized with iPath ( Fig. 2 ) [36] . Figure 2: The effect of niche conditions on the reconstructed metabolic network. Networks were visualized following optimization in ( a ) bulk soil, ( c ) rhizosphere and ( e ) nodule environments. Lines are colour coded based on fitness effect of deleting each reaction: blue indicates a fitness decrease <1%; dark purple indicates a fitness decrease <50%; bright purple indicates a fitness decrease >50%; and red indicates a fitness decrease >99%. Thin grey lines indicate inactive reactions. Line thickness shows the flux through each reaction on a log scale. The graphs summarize the metabolic changes detected during the ( b ) bulk soil to rhizosphere and ( d ) rhizosphere to nodule transitions. Summary of changes graphs: on and off—reactions carrying flux only in the second and first environment, respectively; up and down—reactions carrying increased flux (≥50%) in the second and first environment, respectively; reverse—reactions whose directionality is switched; greater and lesser—reactions whose removal have a greater (≥10%) fitness impact in the second and first environment, respectively; essential and non-essential—reactions essential only in the second and first environment, respectively. The nine classifications are not mutually exclusive. The reactions present in each category are described in Supplementary Data 3 and 4 . The COG analysis graphs summarize the functional annotation of the genes associated with the reactions in the summary of changes graphs. The blue and red bars include the genes associated with the blue and red bars, respectively, in the summary of changes graphs. Asterisks indicate statistically significant changes ( P value <0.01) as determined by Pearson’s χ 2 -tests. In the reaction flux figures, each point represents the amount of flux through individual reactions in the two environments. Blue and purple symbols indicate reactions with the same or reverse directionality, respectively. The angled line indicates the position of a perfect correlation. In the reaction deletion fitness figures, each point represents the fitness of individual reaction deletion mutants in the two environments. The angled line indicates the position of a perfect correlation. Full size image The metabolic network appears globally similar in both the bulk soil and rhizosphere environments ( Fig. 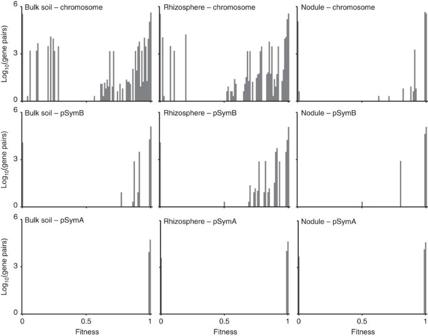Figure 3: Fitness costs associated with double gene deletions in the three tested ecological niches. All possible pairs of genes present on the same replicon were individually removed from the model, the ability of the resulting mutant to produce flux through the objective function was examined with FBA, and the fitness (solution value of the mutant/solution value of the wild type) of each mutant was calculated. The histograms summarize the calculated fitness values for each mutant in each of the three environments separately for each replicon. The fitness is displayed on thexaxis, with the number of mutants displaying that fitness level on theyaxis. The metabolic relevance of a replicon in a particular environment is represented by the number of mutants showing phenotypes between the two extremes (1 and 0); the greater the metabolic relevance, the greater the number of non-extreme phenotypes. 2 and Table 3 ), although many subtle differences were present when reaction specific parameters were examined ( Fig. 2 and Supplementary Data 3 ). Despite good correlation between the log 10 of the absolute flux through a given reaction that was active in both environments ( P value <0.01 using a Spearman’s Rank Order Correlation test, median (absolute residual/observed)=0.09; Supplementary Fig. 5a ), ∼ 20% of the reactions showed at least a 50% change in flux between the two environments while an additional 6% switched directions. Similarly, the effect on fitness (defined as the flux through the objective function (biomass formation or symbiosis) in the mutant relative to the flux through the objective function in the wild type) of individual reaction deletions displayed a strong correlation between the two environments ( P value<0.01 using a Spearman’s Rank Order Correlation test, R 2 =0.95; Supplementary Fig. 5b ). Nevertheless, ∼ 7% had at least a 10% variation in fitness effect between environments, and ∼ 4% were essential in just one of the two niches. Interestingly, optimal growth in the rhizosphere required a greater repertoire of metabolic reaction as illustrated by the increased number of reactions required for maximal fitness. In addition, ∼ 13% of the active reactions were specific to just one of the environments. The reactions whose fluxes were considered to change between growth in bulk soil and the rhizosphere were further validated through a procedure involving flux variability analysis as detailed in Supplementary Note 2 . Table 3 Nutritional composition of the rhizosphere and bulk soil. Full size table Few outstanding biases ( P value <0.01 using a Pearson’s χ 2 -test) were seen in the COG annotations of the genes associated with reactions whose flux or fitness contribution was dependent on the soil environment. This indicated that the reactions important in the rhizosphere were biologically similar to, but functionally distinct from, the reactions important in bulk soil. However, coenzyme transport and metabolism (COG H), and cell wall, membrane and envelope biogenesis (COG M) were more important in the rhizosphere than in the bulk soil. This possibly reflects different coenzyme requirements for the metabolic pathways active in the two environments and the increased succinoglycan content of S. meliloti in the rhizosphere that is necessary to facilitate root biofilm formation. Lipid transport and metabolism (COG I) was over-represented in the bulk soil, perhaps due to the over-abundance of ketogenic amino acids in bulk soil. At the pathway level, only a few changes could not be explained by differences in the nutritional composition and biomass objective functions ( Supplementary Data 3 ). For example, the importance of various carbon catabolic pathways and amino-acid biosynthetic pathways reflected the abundance of the sugars and amino acids in each environment. This analysis also revealed that S. meliloti relies more heavily on glycolytic substrate during growth in bulk soil but on gluconeogenic substrate in the rhizosphere, which was consistent with the high concentration of organic acids in the rhizosphere. The increased gluconeogenic flux and the increased flux through the pantothenate and coenzyme-A biosynthesis pathways in the rhizosphere is also consistent with an increased sugar demand for the rhizosphere-specific Nod factor production and increased exopolysaccharide biosynthesis [37] , [38] . Finally, the urea cycle contributed more to cellular fitness in bulk soil than in the rhizosphere. Complex metabolic reprogramming is associated with symbiosis The rhizosphere to nodule transition was accompanied with much more pronounced metabolic changes than the bulk soil to rhizosphere transition ( Fig. 2 and Supplementary Data 4 ). Half as many reactions carried flux in the nodule than in the rhizosphere, with ∼ 61% of rhizosphere reactions off in the nodule and ∼ 22% of active nodule reactions off in the rhizosphere. This overall decrease in metabolic reactions active in the nodule is consistent with the global transcriptional downregulation in differentiated bacteroids [39] , [40] . For reactions active in both environments, there was a significant correlation ( P value<0.01 using a Spearman’s Rank Order Correlation test; Supplementary Fig. 5c ) in the log 10 of the absolute flux values, but the dispersion of the observed values from the regression line was high (median (residual/observed)=1.48). Approximately half of the common flux carrying reactions displayed at least 50% more flux in one of the environments and a further 12% switched directions. In addition, little correlation was observed between the fitness effects of individual reaction deletions in the two environments ( R 2 =0.03; Supplementary Fig. 5d ). Of the active reactions, ∼ 38% were essential specifically in one environment, while the deletion of another 12% gave fitness effects ≥10% different in the two niches. The reactions whose fluxes were considered to change between growth in the rhizosphere and symbiosis in the nodule were further validated through a procedure involving flux variability analysis as detailed in Supplementary Note 2 . A clear shift in the functional annotation of genes associated with the variable reactions was observed. Functions associated with generating the large amount of energy required for nitrogen fixation displayed increased importance in the nodule: for example, energy production and conversion (COG C), and coenzyme transport and metabolism (COG H). On the other hand, the lack of growth of the differentiated bacteroids not surprisingly rendered biomass component biosynthesis (COGs E, F, L, M, I and J) less important. A few additional interesting observations were noted by looking at pathway level changes ( Supplementary Data 4 ). The Kreb’s cycle and AMP synthesis were increased, presumably to accommodate the high ATP demand of nitrogenase. Glycolysis was less important in the nodule, consistent with the lack of glycolysis-specific enzymes detected in the S. meliloti nodule proteome [41] . Flux through various pathways producing compounds (including steroids, glutathionine, vitamin B6 and haem) required for a successful symbiosis was observed, and in most cases these changes are supported by previously published proteomic, RNA-seq or induction studies [41] , [42] , [43] . Flux through the non-oxidative pentose phosphate pathway, which is poorly studied in S. meliloti [44] , was also increased, consistent with the detection of two enzymes of this pathway in the S. meliloti nodule proteome [41] and the need for S. meliloti to synthesize sugars for biosynthesis [45] . S. meliloti replicons encode niche-specific metabolism We performed comprehensive, replicon-specific in silico single and double gene deletion analyses to determine the contribution of the three S. meliloti replicons to the overall fitness of S. meliloti in each of the tested environments ( Supplementary Table 3 , Fig. 3 and Supplementary Fig. 6 ). The use of a double gene deletion analysis was intended to account for functionally redundancy gene pairs that would mask phenotypes during the single gene deletion analysis [46] , [47] . As before, fitness was determined as the flux through the objective function of the mutant relative to the wild type, with the biomass formation ( Supplementary Table 2 ) being the objective function during growth in bulk soil and the rhizosphere, and N 2 -fixation [19] being the objective function in the nodule environment. Figure 3: Fitness costs associated with double gene deletions in the three tested ecological niches. All possible pairs of genes present on the same replicon were individually removed from the model, the ability of the resulting mutant to produce flux through the objective function was examined with FBA, and the fitness (solution value of the mutant/solution value of the wild type) of each mutant was calculated. The histograms summarize the calculated fitness values for each mutant in each of the three environments separately for each replicon. The fitness is displayed on the x axis, with the number of mutants displaying that fitness level on the y axis. The metabolic relevance of a replicon in a particular environment is represented by the number of mutants showing phenotypes between the two extremes (1 and 0); the greater the metabolic relevance, the greater the number of non-extreme phenotypes. Full size image The mutant analyses revealed that the S. meliloti chromosome had a similar contribution to fitness in bulk soil and the rhizosphere; there was little change in the number of essential or fitness-contributing chromosomal genes in these two environments ( Fig. 3 and Supplementary Table 3 ). However, there was a clear reduction in the importance of the chromosome during symbiosis in the nodule, consistent with microarray data showing that chromosomal genes are over-represented amongst the genes that have low expression levels in the symbiotic bacteria relative to the free-living form [11] . Similar to the chromosome and consistent with the global S. meliloti transcriptional downregulation in the nodule [39] , pSymB contributed more or less only to the fitness of the free-living bacterium, with little role detected in the bacteroids ( Fig. 3 and Supplementary Table 3 ). However, unlike the chromosome, pSymB showed a bias in importance between growth in bulk soil and the rhizosphere; the number of fitness-promoting genes was ∼ 3.5-fold greater in the rhizosphere. Moreover, every pSymB gene that contributed to fitness in bulk soil had a greater fitness contribution in the rhizosphere. This rhizosphere bias was further amplified when considering the origin of fitness-promoting genes. Of the five pSymB genes contributing to fitness in bulk soil, four are involved in arabinose transport or catabolism [48] . All four of these genes have a chromosomal origin and were transferred to pSymB through an inter-replicon translocation event [49] . We therefore detected only a single gene ( smb20201 ) contributing to fitness in bulk soil that originated on pSymB. Similarly, transcriptomics work with the pea symbiont, Rhizobium leguminosarum , indicated that one of its plasmids (pRL8) is over-represented in genes upregulated specifically in the pea rhizosphere [50] . However, with a few exceptions, the fitness contributions of the pLR8 upregulated genes in bulk soil versus the rhizosphere were not determined. Even though these data clearly illustrated that the metabolic capabilities encoded by pSymB are either specific or more important for growth in the rhizosphere than bulk soil, we believe that the observed bias is an under-representation of the actual situation. The succinoglycan biosynthetic genes are classified as essential in both the bulk soil and the rhizosphere due to their inclusion in the biomass objective functions; however, they are not truly essential but likely have greater importance in the rhizosphere through facilitating biofilm formation on the legume root. Furthermore, a more complete formulation of the bulk soil and rhizosphere environment may exaggerate the bias. For example, protocatechuate was not included due to a lack of information on its abundance. However, recent work showed that protocatechuate metabolism improved fitness of R. leguminosarum in the rhizosphere [51] , and 13 pSymB genes are involved in protocatechuate transport and metabolism [52] , [53] . In contrast with the other replicons, the pSymA megaplasmid contributed no fitness-promoting genes ( Fig. 3 and Supplementary Table 3 ). No phenotypes were detected in bulk soil, while the ‘essential’ genes in the rhizosphere were due to the removal of Nod factor biosynthetic genes. In fact, Nod factor biosynthesis is not essential for growth but is required for the initiation of symbiosis. In the nodule, the essential genes that were identified were required for the synthesis and functioning of the nitrogenase enzyme. The lack of fitness-contributing pSymA genes in the nodule was somewhat surprising, although consistent with published data [6] , [54] , perhaps suggesting that few genes outside of the core symbiotic machinery contribute to the nitrogen fixation process. Indeed, the large rearrangements in the structure of pSymA between wild-type S. meliloti nodule isolates [3] may reflect low selective constraints on the pSymA megaplasmid, and thus explain the low metabolic contribution and importance of pSymA even during the symbiotic interaction. The biases observed for the importance of each replicon in the different environments were confirmed via random permutations, testing up to 1,000 different nutritional compositions as described in detail in Supplementary Note 3 . These environments were created by randomly varying, at each iteration, the maximal allowable uptake of each nutrient with respect to the original value and by also randomly removing two nutrients from the environment. Despite some interesting biological insights being derived from this analysis ( Supplementary Note 3 and Supplementary Figs 7 and 8 ), little variation was seen in the number of essential plus fitness-contributing genes on each replicon or in each environment ( Supplementary Figs 7 and 8 ). The robustness of these results to environmental variations provides support for the validity of our conclusions and shows that the niche specialization is not unique to the specific environmental composition used throughout this study. Finally, a comparison of genes differentially contributing to growth in each environment with a recent regulon analysis in S. meliloti [12] was not conclusive due to the low overlap of the data sets ( Supplementary Table 4 and Supplementary Data 5 ; additional details in Supplementary Note 4 ). On the other hand, grouping these genes based on their pangenome classification [12] illustrated that nearly all fitness-contributing genes belonged to the core genome, a clear enrichment relative to the percentage of core genes in iGD1575 overall ( Supplementary Table 5 and Supplementary Data 5 ; additional details in Supplementary Note 5 ). We have completed a comprehensive, manually and experimentally curated genome-scale metabolic reconstruction of a model multipartite genome of the N 2 -fixing endosymbiont S. meliloti , and modelled the metabolic changes associated with niche transition. The switch from bulk soil to the rhizosphere was accompanied by a metabolic fine-tuning, primarily through changes in carbon metabolism and amino-acid biosynthesis. In contrast, moving from the rhizosphere to the nodule involved a comprehensive metabolic reprogramming. This involved essentially shutting off production of all biomass compounds and instead synthesizing co-factors necessary for a successful symbiosis, maximizing ATP production and fixing atmospheric nitrogen. The analysis of the in silico fitness contributions of genes included in iGD1575 revealed that the chromosome is not metabolically specialized for a particular niche, but instead encodes the core metabolic machinery that enables growth of S. meliloti as a free-living microbe. In contrast, the evidence indicated that pSymB is metabolically specialized for the rhizosphere, helping S. meliloti to adapt to this environment and utilize the newly available substrates. The analysis failed to detect any environment where pSymA contributed to improved fitness, but it was seen that pSymA functions were solely relevant to the symbiotic process. Concerning multipartite genome evolution, these observations are consistent with an evolutionary scenario where (1) the gain of pSymB first significantly improved the ability of S. meliloti to colonize the rhizosphere as suggested previously [4] , [55] , (2) pSymB gained additional genes encoding metabolic functions that contribute to fitness predominately in the rhizosphere and (3) pSymA only contributes metabolic functions relevant for establishing a N 2 -fixing symbiosis. We speculate that our observations here with S. meliloti may be generalizable to other bacteria with a multipartite genome that interact with a eukaryotic host. We hypothesize that secondary replicons might facilitate the start of a host interaction; this is the case for the large Escherichia coli virulence plasmids [7] and the rhizobial symbiotic plasmids [18] . Once the organism begins inhabiting the host-associated niche, the secondary replicon might acquire genes that improve fitness specifically in this new environment, whereas the chromosome remains largely undifferentiated, carrying the general metabolic pathways required for life and traits specific to the cell’s original environment. The modelling framework we have developed for this work can be adapted to study other types of biological association (for example, pathogenesis) and the metabolic reprogramming that is needed to operate the switch towards a novel ecological niche. Moreover, by demonstrating here that chromids and megaplasmids carry genes that primarily improve fitness in a specific niche, such as host interaction, this work illustrates secondary replicons as a rich reservoir of genes that have potential in synthetic biology applications. Finally, we anticipate that the iGD1575 model herein reconstructed will represent a valuable platform for future manipulations of S. meliloti aimed at its biotechnological exploitation in the context of agricultural procedures. Metabolic network reconstruction A draft metabolic model was constructed using the KBase Narrative Interface ( www.kbase.us ) and then manually and experimentally validated and expanded based on published data as described in the Supplementary Methods . The final S. meliloti model was termed iGD1575 in accordance with the nomenclature standard [56] , and includes 1,575 genes, 1,825 reactions and 1,579 metabolites. The SBML file of the model was validated by the online SBML validator tool ( http://sbml.org/Facilities/Validator/ ), and is available as Supplementary Data 6 . Metabolic modelling was performed using Matlab R2015a (Mathworks), using scripts from the Cobra Toolbox [57] and the Gurobi 6.0.1 solver ( www.gurobi.com ). A detailed description of the modelling procedure is reported in the Supplementary Methods . For comparison of iGD1575 with previously published flux data [23] , the flux through each reaction was constrained by setting the upper and lower bounds to the average plus or minus the error of the experimentally derived values. To facilitate construction of the in silico large-scale S. meliloti gene deletion mutants in iGD1575, identification of essential model genes was performed as described in Supplementary Note 6 and the essential iGD1575 genes are listed in Supplementary Table 7 . Biomass composition No comprehensive description of the macromolecular composition of the S. meliloti biomass exists in the literature. However, such data are available for Rhodobacter sphaeroides , a related α-proteobacterium [58] . We therefore approximated the S. meliloti gross biomass composition using that of R. sphaeroides . Nevertheless, the specific composition of DNA, RNA, protein and lipids was adjusted based on the S. meliloti GC content [13] , codon usage [59] and lipid composition [60] , [61] , [62] , [63] . Furthermore, succinoglycan was included in the biomass at 5% of the dry weight, which was estimated based on the literature [64] , [65] , [66] . The complete biomass composition is given in Supplementary Table 2 . Objective function formulation The objective function for growth in synthetic media and bulk soil was set as a biomass reaction, producing biomass as described in the above section and fully detailed in Supplementary Table 2 ; this objective function was termed ‘biomass_bulk_c0’. The objective function for growth in the rhizosphere (biomass_rhizo_c0) was the same as for bulk soil except that the amount of succinoglycan was doubled to account for biofilm formation on the plant root, and Nod factor was included (1 mg per g dry weight) as its production would be stimulated by the legume and is required for the initiation of symbiosis ( Supplementary Table 2 ). Finally, the ‘symbiosis_c0’ objective function was adapted from a published S. meliloti model [19] , and was used for modelling symbiosis. In short, the symbiosis objective function involved the synthesis of biomolecules relevant to symbiosis, as well as the export of L -alanine, L -aspartate and ammonium from fixed N 2 . In silico environmental representations In silico representations of the nutritional composition of the rhizosphere and bulk soil were constructed from data available in the literature ( Table 3 ). For both soil representations, ammonium and nitrate were included at a one to one ratio, and sufficient ammonium, nitrate, phosphate, sulphate, metal ions and gases were included so that these compounds were not growth rate limiting. The relative abundance of the major carbon compounds was derived from the available literature as described in the Supplementary Methods . The boundaries of the exchange reactions used to define each environment are listed in Supplementary Table 6 , as are the flux rate through all active exchange reactions. Gene functional analysis The WebMGA webserver [67] was used to provide functional COG annotations ( P value cutoff of 0.001) to each gene in the model. Between-replicon biases were determined after standardizing by the number of genes from each replicon in iGD1575. To perform the COG analyses of the genes associated with variable reactions during the transition between niches, the COG annotation for each gene associated with the variable reaction classes was extracted from the WebMGA output of the previous COG analysis. Biases were determined after standardizing by the number of genes in each class of variable genes. Statistical significance was determined using Pearson’s χ 2 -tests. The complete list of COG annotations is available as Supplementary Data 7 . Phenotype MicroArray analysis Phenotype MicroArray experiments using Biolog plates PM1 and PM2A were performed largely as described previously [25] , [49] with details elaborated on in the Supplementary Methods . All bacterial strains used in this study were described previously [31] , [49] and are listed in Supplementary Table 8 . Of note, whereas most strains were inoculated from agar plates, S. meliloti RmP2754 (ΔB180) and a second wild-type control were inoculated from liquid M9-glucose cultures as RmP2754 grew poorly when inoculated directly from an agar plate. Data analysis was performed with DuctApe [27] . Activity index (AV) values were calculated following subtraction of the blank well from the experimental wells, whereas plots of the growth curves are of the unblanked data. Growth with each compound was considered positive if the AV value was ≥4. Negative growth phenotypes of the mutant strains were called if the AV value was ≤3, and only following manual inspection of the unblanked curves. However, it must be noted that a growth cutoff of 4 is likely to falsely eliminate some compounds that support slow growth of S. meliloti [27] , such as beta-hydroxybutyrate (AV value=3) and acetoacetate (AV value=2) [68] . Growth curves and phosphate determination S. meliloti was grown overnight in LBmc complex medium [4] . These cultures were washed with 0.85% saline and resuspended to an OD 600 of ∼ 0.05 in MM9 minimal medium [4] with either 7.5 mM glucose or 20 mM succinate as the sole carbon source. A volume of 200 μl of the cell suspensions were transferred in triplicate to wells of a 96-well microtitre plates and grown for 24 h at 30 °C with shaking in a BioTek Cytation 3 plate reader. OD 600 readings were measured every 15 min. Growth rates were calculated between OD 600 readings (not corrected for pathlength) of 0.1–0.5 with a previously developed Perl script [4] . To measure the amount of phosphate used by S. meliloti , the phosphate concentrations in the spent media following the completion of the growth curves were determined via the molybdenate blue—ascorbic acid colorimetric method [69] . In brief, cultures were centrifuged, 50 μl of supernatant was diluted with 5 ml of phosphate-free water and 0.8 ml of mixed reagent [69] was added to each sample. Following 10–30 min of incubation at room temperature, the A 880 of each sample was measured and compared with a standard curve. The amount of phosphate remaining in spent media was compared with the phosphate present in the bacteria-free cultures to determine the amount of phosphate used by the bacteria. As the carbon source is growth limiting in these media, the used phosphate to carbon source ratio was calculated by dividing the amount of phosphate removed from the medium by the initial concentration of the carbon source (that is, 7.5 mM glucose or 20 mM succinate). Data availability The authors declare that the data supporting the findings of this study are available within the article and its Supplementary Information files. Matlab scripts used for generation of the FBA data are available from the authors on request. How to cite this article: diCenzo, G. C. et al . Metabolic modelling reveals the specialization of secondary replicons for niche adaptation in Sinorhizobium meliloti . Nat. Commun. 7:12219 doi: 10.1038/ncomms12219 (2016).